Interplay of Dirac fermions and heavy quasiparticles in solids Many-body interactions in crystalline solids can be conveniently described in terms of quasiparticles with strongly renormalized masses as compared with those of non-interacting particles. Examples of extreme mass renormalization are on the one hand graphene, where the charge carriers obey the linear dispersion relation of massless Dirac fermions, and on the other hand heavy-fermion materials where the effective electron mass approaches the mass of a proton. Here we show that both extremes, Dirac fermions, like they are found in graphene and extremely heavy quasiparticles characteristic for Kondo materials, may not only coexist in a solid but can also undergo strong mutual interactions. Using the example of EuRh 2 Si 2 , we explicitly demonstrate that these interactions can take place at the surface and in the bulk. The presence of the linear dispersion is imposed solely by the crystal symmetry, whereas the existence of heavy quasiparticles is caused by the localized nature of the 4 f states. The idea that collective excitations, for example, lattice vibrations, and many-body phenomena, for example, electron correlation, can be described in terms of a rescaled single-particle problem [1] , [2] was a major breakthrough in condensed matter physics. The solutions of such models are quasiparticles that relate the many-body interactions to the properties of a virtual single particle. This concept can provide an understanding of complex phenomena like, for example, the exotic low-temperature physics of heavy-fermion systems—intermetallics synthesized on the basis of 4 f or 5 f elements—where the conduction electrons act as particles with huge masses, comparable to that of a proton [3] , [4] , [5] . The large effective masses are reflected in the low-temperature properties of the material, for instance, by large values of the specific heat or an increase of electric resistivity below the so-called Kondo temperature. In angle-resolved photoemission (ARPES) data, the respective states can be identified as flat running states with an almost complete absence of dispersion. A diametrically opposed example is charge carriers in graphene, which behave as massless Dirac fermions [6] , [7] , [8] , [9] , [10] , which are, like photons, characterized by a linear dispersion relation [8] . The results of A. Geim and K. Novoselov explicitly demonstrate a correlation of this linear dispersion with other unique properties of graphene like the large opacity, the huge charge carrier mobility and the anomalous quantum-Hall effect [6] , [7] , [9] , [10] . Here we report that both extremes, massless and ultra-heavy fermionic quasiparticles may not only coexist in a solid but also even exhibit mutual interaction and form composite quasiparticles. Interaction of a linear dispersive band with localized, that is, ultra-heavy states is used as a text-book example in quantum mechanics to illustrate the mechanism of heavy-fermion formation. Here the localized states lie close to the Fermi level and the interaction leads to weakly dispersive, that is, heavy quasiparticle bands that cross the Fermi level and dominate the low-temperature properties of the materials. Light quasiparticles as derived from the former linear dispersive band do not contribute to the Fermi level region and are, therefore, usually not discussed. To study the latter, we investigated the divalent antiferromagnet (T Neel ~25 K) EuRh 2 Si 2 ( [11] , [12] , [13] ). The isostructural YbRh 2 Si 2 ( [14] , [15] ) and URu 2 Si 2 (ref. 16 ) compounds are famous Kondo-lattice systems where heavy-fermion properties are caused by interaction of f states with transition-element-derived 4 d bands. The homologue system EuIr 2 Si 2 , in spite of its strong fluctuating-valence behaviour, also exhibits remarkable similarities to the latter compounds [17] . It looks so that around the point, the d bands reveal the shape of a Dirac cone that is flattened and slightly deformed by interaction with the f states at the Fermi energy ( E F ). In the stable-valent Eu compound, however, its linear shape survives because the 4 f states and, thus, the related heavy quasiparticle bands are shifted a bit away from the E F . In our ARPES experiments, we observe a conical band with apex close to E F , which passes through an Eu 4 f 6 final-state multiplet and interacts with the latter. The conical shape of respective surface and bulk-derived Rh 4 d bands is properly reproduced by density-functional theory calculations if f–d interaction is suppressed by treating 4 f electrons as core states. The f–d interaction is then introduced within a simple hybridization model and yields linear dispersive, that is, ‘massless’ bands with strong 4 f admixture near E F in coexistence with heavy quasiparticle bands at higher-binding energies in excellent agreement with both surface and bulk-sensitive experiments. ARPES insight into the f–d interaction The linear band dispersion around seems to exist in various members of the tetragonal body-centred ThCr 2 Si 2 (122) family. As it has been already mentioned, in the isostructural Kondo-lattice compound YbRh 2 Si 2 , a respective band has been previously found but there the apex of the Dirac-like cone is slightly deformed by hybridization with 4 f states at the Fermi level [14] , [15] . A similar interplay between heavy 4 f and massless 4 d quasiparticles also occurs in EuRh 2 Si 2 , leading to a pronounced non-crossing behaviour that is explicitly reminiscent to that of polariton generation in optics where a light cone interacts with an almost non-dispersive optical phonon branch [18] . In contrast to YbRh 2 Si 2 , the linear band dispersion is preserved at E F in EuRh 2 Si 2 because of the absence of energetically low-lying 4 f excitations. Because of its hybridization with the 4 f multiplet, the linearly dispersing band accumulates a certain weight of 4 f character, which it carries all the way up to the Fermi-level region. A computational analysis provides a hint to spin polarization of the linear band. This is in close analogy to what is observed for topological insulators [19] , [20] , [21] where respective linear dispersive surface states bridge the band gap and lead to metallic behaviour in the surface layer. However, the linear state in EuRh 2 Si 2 is probably not protected by time-reversal symmetry like in topological insulators because EuRh 2 Si 2 is a metal and the state is also found in the bulk ( Supplementary Fig. S1 ). Thus, it may be closer to the case of graphene where the linear dispersion emerges due to the lattice symmetry. EuRh 2 Si 2 usually cleaves along the Eu layers leaving behind surfaces terminated either by Si or Eu atoms (see Methods and Supplementary Fig. S2 ). In Fig. 1a , we compare the electron band structure as seen by ARPES along the – direction for the two possible surface terminations after cleaving ( Supplementary Note 1 ). The band topologies look rather different in both cases: the 4 f electron emission from bulk Eu atoms, visible as the narrow, string-like 4 f 6 final-state multiplet between 0.2 and 0.8 eV binding energy (BE), is detected for both surfaces, whereas the presence of Eu atoms at the surface gives rise to an additional broad 4 f signal between 1.2 and 2 eV BE. 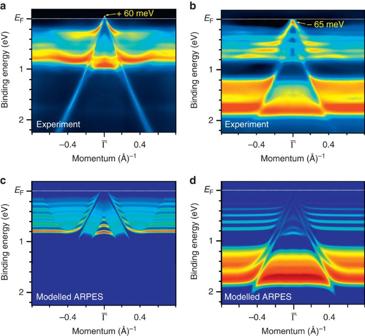Figure 1: Experimental and theoretical insight into the 4f-derived electron structure. ARPES data of (a) Si- and (b) Eu-terminated surfaces are shown in a colour representation where yellow (red) denotes the largest photoemission intensity. The data were taken at 120 eV photon energy, that is, sensitive to 4femissions while signals from Rh 4dstates are strongly suppressed by cross-section effects. Note that Eu termination is concluded from the presence of Eu 4fsurface signals between 1.1 and 1.9 eV BE, whereas the lack of such signals indicates Si termination because the bonding between Si and Rh atoms is tight and cleavage takes place prediominantly between Eu and Si layers (seeSupplementary Fig. S2). Modelled ARPES spectra of respective terminations are presented incandd. Note that only the 4fadmixtures to the bands are plotted, whereas the experimental data reveal weak contributions from states of other symmetries also. Figure 1: Experimental and theoretical insight into the 4 f -derived electron structure. ARPES data of ( a ) Si- and ( b ) Eu-terminated surfaces are shown in a colour representation where yellow (red) denotes the largest photoemission intensity. The data were taken at 120 eV photon energy, that is, sensitive to 4 f emissions while signals from Rh 4 d states are strongly suppressed by cross-section effects. Note that Eu termination is concluded from the presence of Eu 4 f surface signals between 1.1 and 1.9 eV BE, whereas the lack of such signals indicates Si termination because the bonding between Si and Rh atoms is tight and cleavage takes place prediominantly between Eu and Si layers (see Supplementary Fig. S2 ). Modelled ARPES spectra of respective terminations are presented in c and d . Note that only the 4 f admixtures to the bands are plotted, whereas the experimental data reveal weak contributions from states of other symmetries also. Full size image The strong localization of 4 f electrons leads to the observed almost dispersionless behaviour corresponding to the limit of free ions or—rephrased in the band-structure picture—infinitely heavy quasiparticles. These ‘horizontal bands’ are disturbed at those points in k -space, where they are crossed by the linearly dispersing valence band. Where ‘heavy’ and ‘light’ electron bands would cross, the energy degeneracy is lifted by hybridization leading to the formation of small energy gaps and a mixing of the Eu 4 f and Rh 4 d states that is explicitly reflected in the ARPES data. The linear bands clearly hybridize with all J-terms of the Eu 4 f multiplet. The resulting composite states exhibit a non-vanishing f character and are, thus, nicely seen at the chosen photon energy of 120 eV where 4 f emissions dominate. Effectively massless quasiparticles with finite 4 f character appear in this way even at the E F and form a strong contrast to the heavy 4 f- derived quasiparticles usually observed in Kondo systems. Looking closely at the f–d hybrid band, running towards E F in a quasi-conical shape, we can make important observations. The energy position of the cone apex depends on the surface termination: for Si termination, it appears ~60 meV above the Fermi level, whereas for Eu termination, it is located ~65 meV below. Upon changing the photon energy, no notable dispersion in k z direction is observed. These properties are well reproduced in band-structure calculations. To this end, we used a slab geometry where only few atomic layers parallel to the surface are considered, which allows to discriminate between surface and bulk effects. Treating the 4 f electrons as core states, the linearly dispersing bands are reproduced by electron states of almost two-dimensional character, which are located at the surface. Understanding the interaction between localized 4 f and itinerant electrons requires information on the strength of the hybridization, which is intimately related to the symmetry of coupling orbitals. Within a simple hybridization model, one may assume that the hybridization strength is proportional to the f character of the unhybridized valence states at the site of the Eu atoms. Slab-based band-structure calculations and hybridization model The angular momentum character of the valence states may be obtained from the slab calculations ( Supplementary Note 2 ). It can be used then within the hybridization model to simulate the ARPES spectra for both surface terminations of the EuRh 2 Si 2 crystal ( Supplementary Note 3 ). The results are shown in Fig. 1c that qualitatively reproduce the key features of our experimental ARPES data. The linear dispersion of the Rh bands obtained in the slab calculations is mainly preserved in the hybridization model, modified by hybridization gaps and the crossover to the Eu 4 f 6 final-state multiplet. In addition, the hybridization model yields the transfer of Eu 4 f spectral weight to the conically shaped valence band confirming the conclusions drawn from the experimental data. Note that for the calculated spectra in Fig. 1c , only 4 f contribution is shown, whereas in the experimental ARPES spectra, weak contributions from states of other angular momentum character are also visible at the chosen photon energy. In Fig. 2 , we show the unhybridized bulk and surface bands for both surface terminations as computed from the slab model. In the calculations, the localized 4 f states were treated as core states. Green- and blue-dotted lines represent surface bands, which are shifted in energy with respect to the bulk bands, and surface states, which are located inside a bulk band gap, respectively. The thicknesses of these lines scale with the surface to bulk ratio. The bulk band structure projected into the surface Brillouin zone (BZ) [22] is represented by the maroon shading. There is a remarkable agreement between the experimentally derived electron bands and the computed band dispersions for both terminations. In particular, the surface bands with linear dispersion at the point are well reproduced, including the energy difference of the cone apex position between the Eu and Si termination. In addition, there is a finite gap of 200 meV between the upper and the lower cone for both surface configurations. 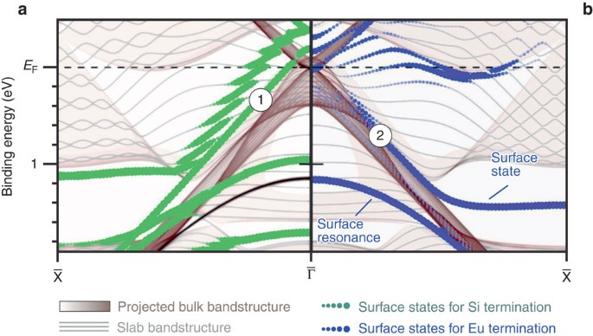Figure 2: Slab-based band-structure calculations. Respective computations were performed for a surface covered by (a) Si and (b) Eu atoms. The maroon-shaded area corresponds to the surface-projected bulk band structure, whereas the grey lines are the result of a calculation for a slab model. The green (blue) dots scale with ratio of localization: if the charge density is mainly located at the surface, then the size of the respective dot is at its maximum, whereas for equally distributed charge density, it vanishes. Figure 2: Slab-based band-structure calculations. Respective computations were performed for a surface covered by ( a ) Si and ( b ) Eu atoms. The maroon-shaded area corresponds to the surface-projected bulk band structure, whereas the grey lines are the result of a calculation for a slab model. The green (blue) dots scale with ratio of localization: if the charge density is mainly located at the surface, then the size of the respective dot is at its maximum, whereas for equally distributed charge density, it vanishes. Full size image Group-theory considerations on two-dimensional lattices show that the quasiparticle dispersion around high-symmetry points is mainly determined by the symmetry of the space group of the crystal lattice [23] , [24] . Similar predictions for the space groups in three dimensions have not been carried out yet, but the arrangement of Rh atoms at the surface in the layered structure of EuRh 2 Si 2 with tetragonal symmetry can up to some extent be approximated by a squared lattice for which in fact the appearance of linear electron dispersion was predicted [23] . The layered character of the compound poses the question whether similar phenomena as observed in the surface region may also be expected for the bulk. The projected bulk band structure shows indeed a band that coincides roughly with the linear surface band and which reveals a weakly three-dimensional (3D) character (dark maroon shading in Fig. 2 ). This becomes more evident in Fig. 3 , where we show cuts at several k z through the bulk BZ, parallel to the – direction. For k z =0.285 π/a, the bands in the vicinity of the point become degenerate and reveal linear dispersion, while for other values of k z , the band dispersions deviate slightly from this linear slope. Thus, similar hybridization phenomena as observed in the surface region may in fact be found in the bulk too. To prove this, we performed an ARPES experiment in the soft X-ray photon-energy range where the photoelectron escape depth is increased and the extreme surface sensitivity of ultraviolet ARPES is partly overcome. 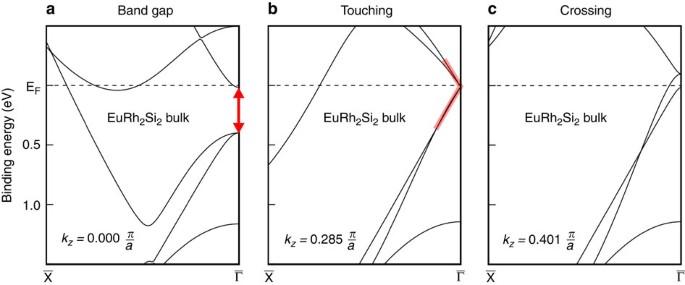Figure 3: Bulk electron band structure. Local density approximation-derived bulk band structure parallel to the–direction for several planes defined by different values ofkz. There are different bands in the region around thepoint close toEF. Going alongkzfrom the centre of the BZ to the top (bottom), one notices that they form a quasi-linear dispersion (two-dimensional) atkz=±0.285 (π/a), which gets enhanced as well as shifted in energy at the surface. Figure 3: Bulk electron band structure. Local density approximation-derived bulk band structure parallel to the – direction for several planes defined by different values of k z . There are different bands in the region around the point close to E F . Going along k z from the centre of the BZ to the top (bottom), one notices that they form a quasi-linear dispersion (two-dimensional) at k z =±0.285 (π/a), which gets enhanced as well as shifted in energy at the surface. Full size image In Fig. 4 , we show an ARPES map of EuRh 2 Si 2 taken at hv =950 eV that extends over the points of three adjacent Brillouin zones. As we know from respective results for the isostructural compound YbRh 2 Si 2 ( [25] ), the contribution of the first subsurface Eu layer amounts to about only 20% of the total 4 f emission at this photon-energy range, whereas it amounts to about 60% in the data shown in Fig. 1 . In fact, scanning the beam across the whole surface of freshly cleaved EuRh 2 Si 2 , we did not detect a sign of surface-related electron states. In particular, we never found the surface Eu 4 f feature at ~1.6 eV BE, although the atomic cross-section for Rh 4 d and Eu 4 f is of the same magnitude at 950 eV photon energy. In the ultraviolet photon-energy range, it was always seen for some regions of the sample surface. The absence of surface-related features confirms the high bulk sensitivity in the soft X-ray range. In the region around the points, we observe well-defined bands that approach E F in a quasi-linear way similar to the surface band discussed above. Furthermore, we also detect the string-like Eu 4 f 6 final-state multiplet, which again hybridizes with the linearly dispersive bands. The strong similarities between the surface-sensitive extreme ultraviolet and the more bulk-sensitive soft X-ray data are because of the layered structure of the material and the weak 3D character of the underlying Rh 4 d band. Although the energy and momentum resolution in the soft X-ray range are not as high as in the extreme ultraviolet, they still allow the conclusion that ultra-light and heavy quasiparticles coexist for particular cuts through the 3D Brillouin zone of the material too, and are subjected to the same hybridization phenomena as their surface counterparts. 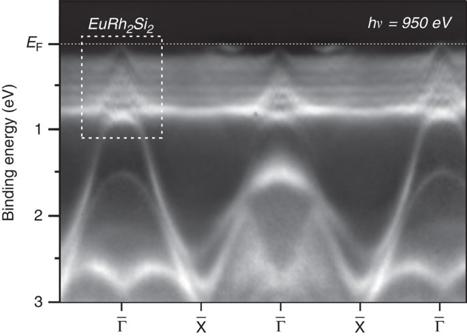Figure 4: Insight into the bulk electronic structure. Experimental ARPES data of EuRh2Si2recorded using 950 eV photons, which allows to suppress the emission from the surface states and thus to disentangle the bulk electron structure of the system. The dotted frame shows the region where conically shaped Rh bands with their apex close to the Fermi level are coupled with a bunch of ‘horizontal’ bands from the bulk Eu 4f6multiplet. Figure 4: Insight into the bulk electronic structure. Experimental ARPES data of EuRh 2 Si 2 recorded using 950 eV photons, which allows to suppress the emission from the surface states and thus to disentangle the bulk electron structure of the system. The dotted frame shows the region where conically shaped Rh bands with their apex close to the Fermi level are coupled with a bunch of ‘horizontal’ bands from the bulk Eu 4 f 6 multiplet. Full size image In summary, we have demonstrated that massless and heavy-fermion quasiparticles may not only coexist but can also strongly interact in solids. Applying ultraviolet and soft X-ray ARPES on EuRh 2 Si 2 single crystals, we observed linearly dispersing Rh 4 d -derived bands, corresponding to massless Dirac quasiparticles. Their conical shape is mainly imposed by the in-plane square symmetry of the layered compound. These linear bands are interfered by flat, dispersionless Eu 4 f states corresponding to quasiparticles with extremely large effective masses. At the regions of intersection of both kinds of bands, hybridization gaps as well as strong admixture of the 4 f electron states to the Dirac fermions are detected. This unambiguously demonstrates a strong interplay between these two opposing limits of mass-renormalized fermions. Similar observations as for the surface were made for the bulk of the crystal. Because the symmetry of the layered (122) compounds dictates the formation of ultra-light quasiparticles, one may anticipate that details of their interactions with 4 f states could have a role in the emergence of unusual thermodynamic properties like Kondo physics or quantum criticality in other compounds of this family. Experiment All the ARPES experiments were performed at the Swiss Light Source facility. The surface-sensitive ultraviolet spectra (ultraviolet ARPES) were obtained at the Surface/Interface: Spectroscopy (SIS) instrument, whereas for probing the truly bulk-derived electronic structure, the respective experiments were conducted in the soft X-ray regime (soft X-ray ARPES) at the novel Advanced Resonant Spectroscopies (ADRESS) station. The ultraviolet ARPES spectra were taken using a VG-Scienta R4000 electron analyzer, and SX-ARPES spectra were acquired with a Phoibos 150 machine (Specs GmbH). For both types of experiments, high-quality single crystals of EuRh 2 Si 2 were mounted on a low-temperature goniometric manipulator (CARVING) with three angular degrees of freedom and cleaved in situ in ultra-high vacuum with a base pressure better than 5 × 10 −11 mBar at T =10 K. Subsequently, the cleaved samples were explored with the aforementioned photoemission approaches, keeping them at the same temperature. The time scheduled for studying each sample was about 4 h, including crystal alignment. Sample preparation Single crystals of EuRh 2 Si 2 were grown in indium flux as described in Seiro and Geibel [11] . Excess flux was removed by chemical etching with diluted HCl, yielding 1–5 -mm wide flat platelets with the crystallographic c axis along the thin (<1 mm) dimension. EuRh 2 Si 2 crystallizes in the I4/mmm tetragonal structure and orders antiferromagnetically below 24.8 K (refs 11 , 12 ). The Sommerfeld coefficient of the specific heat is roughly 25 mJ K −2 mol ( [11] ), well below that observed for heavy-fermion materials. Theory The calculations have been performed with a density-functional theory code based on the full-potential local orbital method [26] . Unless otherwise stated, the local density approximation in the formulation of Perdew–Wang and the scalar-relativistic approximation was employed. The 4 f electrons were treated as core states (see Supplementary Note 2 ) using an unpolarized configuration close to experiment. The slab configurations to simulate the surface have been constructed in such a way that the original centrosymmetry was preserved. For k -space sampling, at least 144 k II points in the surface Brillouin zone were taken into account. The differentiation in surface and bulk states has been achieved by comparing the localization of the Bloch eigenfunctions. How to cite this article: Höppner, M. et al . Interplay of Dirac fermions and heavy quasiparticles in solids. Nat. Commun. 4:1646 doi: 10.1038/ncomms2654 (2013).